TOPLESS mediates brassinosteroid-induced transcriptional repression through interaction with BZR1 Brassinosteroid (BR) regulates plant development by activating the transcription factor brassinazole resistant 1 (BZR1), which activates and represses different target genes to switch cellular programmes. The mechanisms that determine BZR1’s transcriptional activities remain largely unknown. Here we show that BZR1 represses target genes by recruiting the Groucho/TUP1-like transcriptional corepressor TOPLESS (TPL). Specific deletion or mutation of an evolutionarily conserved ERF-associated amphiphilic repression (EAR) motif at the carboxy terminus abolishes BZR1’s abilities to regulate gene expression and cell elongation, but these defects are rescued by TPL fusion to the EAR motif-mutated BZR1. The EAR motif in BZR1 mediates recruitment of TPL to BZR1-repressed promoters. A triple tpl mutant ( tpl;tpr1;tpr4 ) shows reduced BR sensitivity and suppresses the gain-of-function bzr1-1D mutant phenotype. BR repression of gene expression also requires histone deacetylases that interact with TPL. Our study demonstrates key roles of the EAR motif and TPL in BR regulation of gene expression and plant growth. Steroids are important hormones for regulation of gene expression and development in both animals and plants. Unlike animal steroid hormones, which directly bind to nuclear receptor transcription factors, the plant steroid hormone brassinosteroid (BR) binds to a transmembrane receptor kinase, brassinosteroid insensitive1 (BRI1) [1] , which has a leucine-rich repeat extracellular domain similar to the Toll receptors in metazoans [2] . BRI1 signalling activates the members of the brassinazole resistant1 (BZR1) family of transcription factors through a phosphorylation-mediated signal transduction pathway [3] , [4] . BZR1 activates and represses different target genes to programme genome expression and cell growth. The mechanisms that specify BZR1’s function in transcription activation and repression are not understood. BZR1 is a plant-specific transcription factor with a DNA-binding domain that recognizes BR response element (CGTG(T/C)G) [5] . Both subcellular localization and DNA-binding activity of BZR1 are tightly regulated by phosphorylation. In the absence of BR, a glycogen synthase kinase 3 (GSK3)-like kinase named BIN2 interacts with BZR1 via a docking motif at the C terminus of BZR1 and phosphorylates BZR1 (refs 6 , 7 , 8 ). The phosphorylated BZR1 is unable to bind DNA and also is retained in the cytosol due to binding to the 14-3-3 proteins [9] , [10] . BR binding to BRI1 triggers a signalling cascade that leads to inactivation of BIN2 (ref. 11 ), resulting in dephosphorylation of BZR1 catalysed by protein phospatase 2A (PP2A) [12] . Dephosphorylated BZR1 enters the nucleus and binds to target promoters to mediate BR-responsive gene expression [3] . BZR2 (also named BES1), the close homologue of BZR1, is regulated through similar mechanisms [6] , [12] , [13] , [14] . Similar to many plant transcription factors, BZR1 functions as a transcriptional repressor for some promoters but an activator for others. Previous genome-wide identification of direct binding sites of BZR1 coupled with transcriptome profiling showed that BZR1 binds to promoters of both BR-repressed and -induced genes [5] , [15] . Apparently, BZR1 transcriptional activity is partly determined by the context of promoter cis -elements and trans -factors. Indeed the genome-wide data showed that BR response element is enriched in the promoters of BR-repressed gene, whereas the E-box motif (CANNTG), a binding site for bHLH factors, is more enriched in the promoters of BR-activated genes [15] . BZR1 and its homologous BZR2/BES1 interact with the bHLH factor phytochrome interacting factor4 (PIF4) and BZR1 shares with PIF4 over 50% of their target genes in the genome. BZR2/BES1 also interacts with BES1-interacting Myc-like1 (BIM1). The BZR1-PIF4 and BZR2-BIM1 heterodimers bind to the E-box motif in the promoters of target genes and activate gene expression [13] , [16] . Several other transcription factors and histone-modifying enzymes have been reported to interact with BZR2/BES1 and participate in BZR2/BES1 activation of gene expression [17] , [18] , [19] . In addition, recent studies have suggested that myeloblastosis transcription factor like2 (MYBL2) and homeodomain-leucine zipper protein1 (HAT1) interact with BZR2/BES1 and repress several BR target genes [20] , [21] . However, it remains unclear how BZR1 represses gene expression, and specifically how its gene repression and activation activities are mediated by interactions with general transcriptional regulators. In this study, a genetic screen for the intragenic suppressors of the gain-of-function mutant bzr1-1D reveals an important function of an evolutionarily conserved ERF-associated amphiphilic repression (EAR) motif in BZR1 regulation of target gene expression. We further show that BZR1 EAR motif mediates interaction with the Groucho/TUP1-like corepressor TOPLESS (TPL), selectively recruiting TPL to the promoters of BZR1-repressed target genes. BZR1 repression of gene expression requires both TPL and also the activity of histone deacetylase (HDA) that is known to interact with TPL. Our study unveils the molecular mechanism of BR repression of gene expression through BZR1–TPL interaction. EAR motif is crucial for BZR1 functions The gain-of-function mutant BZR1 protein, bzr1-1D, is constitutively dephosphorylated and active even in the BR deficiency condition due to a strong interaction with PP2A [12] . Thus, the hypocotyl elongation of bzr1-1D seedling is resistant to BR biosynthesis inhibitors, brassinazole (BRZ) and propiconazole (PPZ) [12] . We identified suppressors of the bzr1-1D mutant through an EMS mutagenesis screen. One of the mutants, bzs285 , carried a mutation that creates a stop codon after amino acid 284, resulting in deletion of 52 amino acids at the C terminus of bzr1-1D protein ( Fig. 1a,b ). The truncated region includes a BIN2 docking motif and an LxLxL type of EAR motif. As the BIN2 docking motif mediates inactivation of BZR1 through BIN2-mediated phosphorylation [8] , the suppression of the bzr1-1D phenotype by the bzs285 mutation was most likely to be due to the loss of the EAR motif. The EAR motif is highly conserved in the BZR1 family of transcription factors across land plants from bryophytes to angiosperms ( Supplementary Fig. 1a ). In addition, all other BZR1-like proteins in Arabidopsis have the EAR motif at their C terminus ( Supplementary Fig. 1b ), implicating an indispensable role of the EAR motif in BZR1 functions. 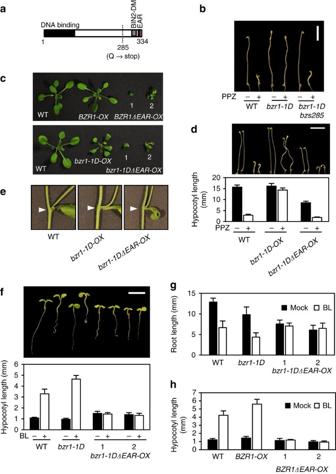Figure 1: EAR motif is essential for BZR1 function in BR responses. (a) Glutamine (Q) at position 285 in BZR1 is converted to stop codon in thebzs285mutant. BIN2-DM: BIN2 docking motif; EAR: EAR motif. (b) Intragenic mutant (bzs285) suppresses the constitutive activation of BR response ofbzr1-1D. Seedlings were grown in the dark on the medium containing 2 μM PPZ. Scale bar, 5 mm. (c) BothBZR1ΔEAR-OXsandbzr1-1DΔEAR-OXsshow severe dwarfism. Plants were grown in the long-day condition (16 h of light and 8 h of dark) for 4 weeks. Two independent lines (1 and 2) for theBZR1ΔEAR-OXsandbzr1-1DΔEAR-OXsare shown. (d) The hypocotyl elongation ofbzr1-1DΔEAR-OXis inhibited by PPZ treatment. Seedlings were grown in the dark for 5 days on the medium containing either the mock or 2 μM PPZ. Error bars indicate the s.d. (n=10 plants). Scale bar, 5 mm. (e) Axillary branches and cauline leaves are not fused inbzr1-1DΔEAR-OX.(f,g)bzr1-1DΔEAR-OXsare insensitive to BR in the promotion of hypocotyl elongation (f) and the inhibition of primary root growth (g). Seedlings were grown under the white light for 5 days on the medium containing either mock or 1,000 nM brassinolide (BL). Scale bar, 5 mm. (h)BZR1ΔEAR-OXsare insensitive to BR in the promotion of hypocotyl elongation. Seedlings were grown under the white light for 5 days on the medium containing either mock or 1,000 nM brassinolide (BL). Error bars in (f–h) indicate the s.d. (n=10 plants). Figure 1: EAR motif is essential for BZR1 function in BR responses. ( a ) Glutamine (Q) at position 285 in BZR1 is converted to stop codon in the bzs285 mutant. BIN2-DM: BIN2 docking motif; EAR: EAR motif. ( b ) Intragenic mutant ( bzs285 ) suppresses the constitutive activation of BR response of bzr1-1D . Seedlings were grown in the dark on the medium containing 2 μM PPZ. Scale bar, 5 mm. ( c ) Both BZR1ΔEAR-OXs and bzr1-1DΔEAR-OXs show severe dwarfism. Plants were grown in the long-day condition (16 h of light and 8 h of dark) for 4 weeks. Two independent lines (1 and 2) for the BZR1ΔEAR-OXs and bzr1-1DΔEAR-OXs are shown. ( d ) The hypocotyl elongation of bzr1-1DΔEAR-OX is inhibited by PPZ treatment. Seedlings were grown in the dark for 5 days on the medium containing either the mock or 2 μM PPZ. Error bars indicate the s.d. ( n =10 plants). Scale bar, 5 mm. ( e ) Axillary branches and cauline leaves are not fused in bzr1-1DΔEAR-OX. ( f , g ) bzr1-1DΔEAR-OXs are insensitive to BR in the promotion of hypocotyl elongation ( f ) and the inhibition of primary root growth ( g ). Seedlings were grown under the white light for 5 days on the medium containing either mock or 1,000 nM brassinolide (BL). Scale bar, 5 mm. ( h ) BZR1ΔEAR-OXs are insensitive to BR in the promotion of hypocotyl elongation. Seedlings were grown under the white light for 5 days on the medium containing either mock or 1,000 nM brassinolide (BL). Error bars in ( f – h ) indicate the s.d. ( n =10 plants). Full size image To functionally characterize the EAR motif of BZR1, we generated transgenic plants overexpressing the EAR motif-deleted BZR1 ( BZR1ΔEAR-OX ) or bzr1-1D ( bzr1-1DΔEAR-OX ). Transgenic plants overexpressing wild-type BZR1 ( BZR1-OX ) were almost indistinguishable from wild-type plants ( Fig. 1c ) due to posttranslational regulation of BZR1 activity by BIN2, whereas overexpression of bzr1-1D ( bzr1-1D-OX ) caused BR-activation phenotypes similar to the bzr1-1D mutant ( Fig. 1c ), including leaf bending, organ fusion, and insensitivity to BR inhibitors [22] . In contrast, both BZR1ΔEAR-OX and bzr1-1DΔEAR-OX plants displayed severe dwarfism ( Fig. 1c ), similar to the BR-insensitive or BR-deficient mutant plants, suggesting that the EAR-deleted BZR1 proteins have dominant negative effects on BR responses. Consistent with bzr1-1D suppression by bzs285 , bzr1-1DΔEAR-OX plants were sensitive to BR biosynthetic inhibitor PPZ ( Fig. 1d ) and showed no organ-fusion phenotypes in contrast to the fusion between cauline leaves and axillary branches often observed in the bzr1-1D and bzr1-1D-OX plants [22] ( Fig. 1e ). The bzr1-1DΔEAR-OX seedlings grown in the dark also showed shorter hypocotyls ( Fig. 1d ). These results confirm an essential role of the EAR motif in BZR1 function. To determine whether the dwarfism is caused by a defect in BR signalling or BR biosynthesis, we examined BR response of the bzr1-1DΔEAR-OX . Although the hypocotyls of bzr1-1D were more elongated by BR treatment than those of wild type, hypocotyls of bzr1-1DΔEAR-OX were insensitive to BR ( Fig. 1f ), indicating that BR signalling is impaired in the bzr1-1DΔEAR-OX plants. BR inhibits primary root growth mainly through reducing cell division in the root meristem [23] . Root growth of bzr1-1D was more sensitive to BR inhibition than wild type, whereas roots of the bzr1-1DΔEAR-OX were insensitive to BR ( Fig. 1g ). Similar to bzr1-1DΔEAR-OXs , BZR1ΔEAR-OXs also showed BR insensitivity in hypocotyl elongation ( Fig. 1h ). The severe dwarfism and BR insensitivity of BZR1ΔEAR-OX and bzr1-1DΔEAR-OX are most likely to be due to the dominant negative effects of the EAR motif-deleted BZR1 over endogenous BZR1 and BZR1-like transcription factors. Together, these results demonstrate that the EAR motif is essential for BZR1 functions in various BR responses. EAR motif mediates BZR1 regulation of gene expression We next analysed the effects of the EAR motif deletion on BZR1 regulation of target gene expression. BZR1 is known to directly repress BR biosynthesis genes, including DWF4 and CPD , to provide the feedback regulation of BR level [5] . The expression levels of DWF4 and CPD were dramatically reduced in bzr1-1D compared with wild type, but was only marginally reduced in the bzr1-1DΔEAR-OX plants ( Fig. 2a ), indicating that the transcriptional repression activity is impaired in bzr1-1DΔEAR. BZR1 also activates expression of many of its target genes [15] . Although the expression levels of SAURs , IAA19 and PRE5 were highly increased by bzr1 - 1D , the expression of SAUR19 , IAA19 and PRE5 was not activated, and SAUR15 expression was only slightly activated by bzr1-1DΔEAR ( Fig. 2b ), suggesting that the EAR motif is also required for the BZR1-mediated transcriptional activation of target genes. 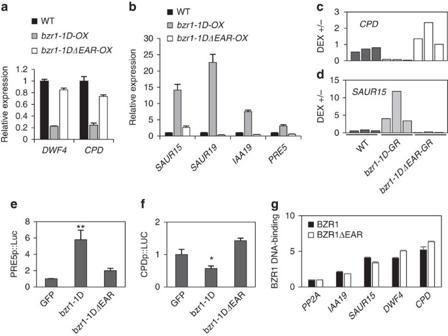Figure 2: EAR motif mediates BZR1 regulation of gene expression. (a,b) The deletion of EAR motif abolishes BZR1 regulation of gene expression. Seedlings were grown on the medium containing 2 μM PPZ in the dark for 5 days before harvesting for RNA extraction. Gene expression levels are normalized to that ofPP2Aand are shown relative to the expression levels in wild type (Col-0). (c,d) The EAR motif-deleted bzr1-1D neither repressesCPDexpression (c) nor activatesSAUR15expression (d). Four-week-old leaves of transgenic plants expressingbzr1-1D-GRorbzr1-1DΔEAR-GRwere treated with mock or 40 μM of dexamethasone (DEX) for 4 h. Ratios of expression levels in DEX-treated to mock-treated are shown. Each bar represents independent transgenic plant. (e,f) The EAR motif-deleted bzr1-1D cannot activatePRE5promoter activity (e) and cannot repressCPDpromoter activity (f) in a transient gene expression assay. The 2 kb ofPRE5promoter or 1 kb ofCPDpromoter fused to firefly luciferase reporter gene was co-transfected with35S::bzr1-1Dor35S::bzr1-1DΔEARintoArabidopsismesophyll protoplast. The firefly luciferase activities were normalized byRenillaluciferase as an internal control and are shown relative to that of protoplasts transfected with35S::GFP(GFP). **P<0.01 and *P<0.05 by Student’st-test. (g) The deletion of EAR motif does not affect BZR1 DNA binding. Transgenic plants overexpressingBZR1andBZR1ΔEARwere treated with 100 nM BL and cross-linked for the ChIP assays. In the ChIP assays, the enrichment of DNA was calculated as the ratio between transgenic plants and wild-type control (Col-0), normalized to that of thePP2Acoding region as an internal control. Error bars in (a,b,e,f,g) indicate the s.d. (n=3). Figure 2: EAR motif mediates BZR1 regulation of gene expression. ( a , b ) The deletion of EAR motif abolishes BZR1 regulation of gene expression. Seedlings were grown on the medium containing 2 μM PPZ in the dark for 5 days before harvesting for RNA extraction. Gene expression levels are normalized to that of PP2A and are shown relative to the expression levels in wild type (Col-0). ( c , d ) The EAR motif-deleted bzr1-1D neither represses CPD expression ( c ) nor activates SAUR15 expression ( d ). Four-week-old leaves of transgenic plants expressing bzr1-1D-GR or bzr1-1DΔEAR-GR were treated with mock or 40 μM of dexamethasone (DEX) for 4 h. Ratios of expression levels in DEX-treated to mock-treated are shown. Each bar represents independent transgenic plant. ( e , f ) The EAR motif-deleted bzr1-1D cannot activate PRE5 promoter activity ( e ) and cannot repress CPD promoter activity ( f ) in a transient gene expression assay. The 2 kb of PRE5 promoter or 1 kb of CPD promoter fused to firefly luciferase reporter gene was co-transfected with 35S::bzr1-1D or 35S::bzr1-1DΔEAR into Arabidopsis mesophyll protoplast. The firefly luciferase activities were normalized by Renilla luciferase as an internal control and are shown relative to that of protoplasts transfected with 35S::GFP (GFP). ** P <0.01 and * P <0.05 by Student’s t -test. ( g ) The deletion of EAR motif does not affect BZR1 DNA binding. Transgenic plants overexpressing BZR1 and BZR1ΔEAR were treated with 100 nM BL and cross-linked for the ChIP assays. In the ChIP assays, the enrichment of DNA was calculated as the ratio between transgenic plants and wild-type control (Col-0), normalized to that of the PP2A coding region as an internal control. Error bars in ( a , b , e , f , g ) indicate the s.d. ( n =3). Full size image To more directly examine the functions of the EAR motif in BZR1 regulation of gene expression, we generated transgenic plants expressing bzr1-1D or bzr1-1DΔEAR fused to the glucocorticoid receptor (GR), bzr1-1D-GR or bzr1-1DΔEAR-GR , which allows inducible nuclear localization of the fusion proteins. Transient DEX treatment (4 h) of the bzr1-1D-GR plants dramatically repressed CPD expression and activated SAUR15 expression, confirming the inducible nuclear localization and function of bzr1-1D-GR in planta ( Fig. 2c,d ). In contrast, the DEX treatment of the bzr1-1DΔEAR-GR plants did not repress CPD or activate SAUR15 ( Fig. 2c,d ), indicating that the EAR motif is necessary for both transcriptional repression and activation activities of BZR1. In fact, the CPD expression levels were slightly increased by DEX treatment in bzr1-1DΔEAR-GR plants ( Fig. 2c ), most likely to be due to the competition by the transcriptionally inactive bzr1-1DΔEAR protein with the endogenous BZR1 for target promoter occupancy. Consistent with the results of the DEX treatment assays, in transient gene expression assays using Arabidopsis mesophyll protoplasts, bzr1-1D increased PRE5 promoter activity and decreased DWF4 promoter activity, whereas bzr1-1D Δ EAR could neither activate PRE5 nor repress DWF4 ( Fig. 2e,f ). The deletion of the EAR motif did not affect the BZR1 binding to the promoters of target genes ( Fig. 2g ). These results indicate that the deletion of the EAR motif abolishes both gene repression and activation functions of BZR1. To examine the possibility that the deletion of the EAR motif affects the phosphorylation of BZR1, we checked the phosphorylation status of BZR1 and BZR1ΔEAR before and after BR treatment. Wild-type BZR1 protein was mostly phosphorylated when seedlings were grown on the medium containing PPZ and dephosphorylated after BR treatment, but BZR1ΔEAR was highly dephosphorylated even without BR treatment ( Supplementary Fig. 2a ). Such high level of dephosphorylated BZR1ΔEAR is likely to be responsible for the strong phenotypes of BZR1ΔEAR-OX plants in contrast to the lack of phenotype of BZR1-OX plants ( Fig. 1 ). As the EAR motif is located near the BIN2-docking motif [8] , it is likely to be that the deletion of the EAR motif affects BZR1–BIN2 interaction. However, BZR1ΔEAR still interacted with BIN2 in a yeast two-hybrid assay ( Supplementary Fig. 2b ). Moreover, the endogenous BZR1 was also partially dephosphorylated before BR treatment in the BZR1ΔEAR-OX plants ( Supplementary Fig. 2a ), suggesting that BR signalling upstream of BZR1 is activated in the BZR1ΔEAR-OX plants, most likely to be due to the loss of the feedback inhibition of BR synthesis and upstream BR signalling. Indeed, quantitative reverse transcription–PCR (qRT–PCR) analysis showed that the expression level of BIN2 is decreased in bzr1-1DΔEAR-OX compared with that in wild type ( Supplementary Fig. 2c ), which probably contributes to the decreased BZR1 phosphorylation. SRDX fusion restores the functions of EAR motif-deleted BZR1 An EAR motif-based artificial transcriptional repression domain (LDLDLELRLGFA), named SRDX, confers a dominant transcriptional repression activity to the linked transcription factor and has been widely used in functional studies of transcription factors in plants [24] . To determine whether SRDX provides the same function as the EAR motif in BZR1, we generated transgenic plants overexpressing bzr1-1DΔEAR fused with SRDX at the C terminus ( bzr1-1DΔEAR-SRDX-OX ) ( Fig. 3a ). On the medium containing PPZ, the hypocotyls of wild type and bzr1-1DΔEAR-OX were much shorter than that of bzr1-1D , indicating the inability of bzr1-1DΔEAR to promote hypocotyl elongation ( Fig. 3b ). In contrast, bzr1-1DΔEAR-SRDX-OX had much longer hypocotyl than wild type ( Fig. 3b ). In addition, the SRDX fusion restored the BR sensitivity of bzr1-1DΔEAR-OX in the inhibition of primary root growth ( Fig. 3c ), indicating that the functions of EAR motif can be replaced by SRDX. 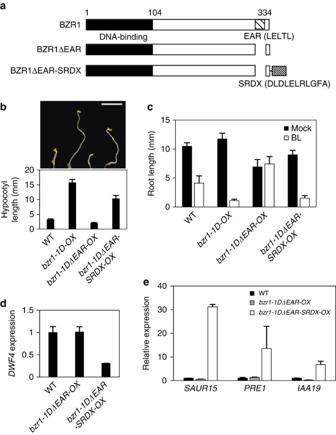Figure 3: SRDX fusion restores the functions of EAR motif-deleted BZR1. (a) Box diagram of BZR1, BZR1ΔEAR and BZR1ΔEAR-SRDX. (b,c) SRDX fusion restores both BZR1 promotion of hypocotyl elongation and inhibition of primary root growth. Seedlings were grown in the dark for 5 days on the medium containing 2 μM PPZ (b) or grown under light for 5 days on the medium containing either mock or 1,000 nM BL (c). The error bars indicate the s.d. (n=10 plants). Scale bar, 5 mm. (d,e) qRT–PCR analyses of BZR1-regulated genes. RNA was extracted from seedlings grown in the dark for 5 days on the medium containing 2 μM PPZ. Gene expression levels are normalized to that ofPP2Aand are shown relative to the expression levels in wild type. The error bars indicate the s.d. (n=3). Figure 3: SRDX fusion restores the functions of EAR motif-deleted BZR1. ( a ) Box diagram of BZR1, BZR1ΔEAR and BZR1ΔEAR-SRDX. ( b , c ) SRDX fusion restores both BZR1 promotion of hypocotyl elongation and inhibition of primary root growth. Seedlings were grown in the dark for 5 days on the medium containing 2 μM PPZ ( b ) or grown under light for 5 days on the medium containing either mock or 1,000 nM BL ( c ). The error bars indicate the s.d. ( n =10 plants). Scale bar, 5 mm. ( d , e ) qRT–PCR analyses of BZR1-regulated genes. RNA was extracted from seedlings grown in the dark for 5 days on the medium containing 2 μM PPZ. Gene expression levels are normalized to that of PP2A and are shown relative to the expression levels in wild type. The error bars indicate the s.d. ( n =3). Full size image Consistent with the established SRDX function, the SRDX fusion restored the transcriptional repression activity of bzr1-1DΔEAR as shown by downregulation of DWF4 expression in the bzr1-1DΔEAR-SRDX-OX plants ( Fig. 3d ). However, to our surprise, bzr1-1DΔEAR-SRDX also activated expression of SUAR15 and IAA19 ( Fig. 3e ), which are direct targets of BZR1, suggesting that SRDX also mediates the transcriptional activation function of BZR1. BZR1 interacts with TPL through the EAR motif In several transcription factors, the EAR motif has been known to mediate transcriptional repression through interaction with TPL and the homologous TPL-related (TPR) proteins [25] , [26] , [27] , [28] . Our recent tandem affinity purification of BZR1 complex followed by mass spectrometry analysis suggested that TPL associates with BZR1 in vivo [29] . We therefore tested whether BZR1 directly interacts with TPL and TPRs. Indeed, in the yeast two-hybrid assay, BZR1 interacted with TPL and also other TPRs ( Fig. 4a,c ). Deletion of the EAR motif or mutation of the conserved Leu residues in the EAR motif abolished the BZR1–TPL interaction ( Fig. 4a,b ), indicating that BZR1 interacts with TPL through the EAR motif. To confirm the BZR1–TPL interaction in vivo , we performed co-immunoprecipitation (co-IP) assays using Arabidopsis mesophyll protoplasts expressing bzr1-1D-GFP or bzr1-1DΔEAR-GFP and TPL-Myc. The TPL-Myc protein was co-immunoprecipitated by anti-YFP antibody specifically when bzr1-1D-GFP was co-expressed ( Fig. 4d ), confirming the in vivo BZR1–TPL interaction. The deletion of EAR motif greatly reduced the TPL–BZR1 interaction in vivo ( Fig. 4d ), which is consistent with the result of the yeast two-hybrid assay ( Fig. 4a ). Thus, both yeast two-hybrid and co-IP assays demonstrate that BZR1 interacts with TPL through the EAR motif. 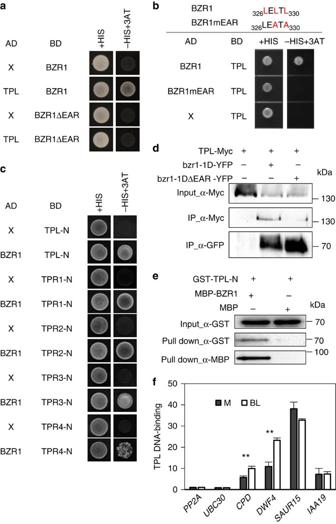Figure 4: BZR1 interacts with TOPLESS through the EAR motif. (a) A yeast two-hybrid assay shows the interaction between BZR1 and TPL. Yeast clones were grown on the synthetic dropout (+His) or synthetic dropout without histidine (-His) plus 50 mM 3AT medium. (b) Mutation in the EAR motif abolishes the BZR1–TPL interaction. Core Leu residues of the EAR motif were substituted to Ala. Yeast clones were grown on the synthetic dropout (+His) or synthetic dropout without histidine (−His) plus 1 mM 3AT medium. (c) BZR1 interacts with TPL and other TPRs. Yeast clones were grown on the synthetic dropout (+His) or synthetic dropout without histidine (−His) plus 5 mM 3AT medium. TPL-N, N-terminal domain of TPL (1–344); TPR1-N, 1–343; TPR2-N, 1–335; TPR3-N, 1–335; and TPR4-N, 1–344. (d) BZR1 interacts with TPL through EAR motifin vivo.Arabidopsismesophyll protoplasts were transfected withTPL-Myctogether withbzr1-1D-GFPorbzr1-1DΔEAR-GFP, and the extracted proteins were immunoprecipitated by anti-GFP antibody. Gel blots were probed with anti-Myc or anti-GFP antibody. (e) TPL binds toDWF4promoter through BZR1. GST-TPL-N (amino acids 1–344) was incubated with a biotin-labelledDWF4promoter DNA (400 bps) together with MBP or MBP-BZR1 and pulled down with streptavidin agarose beads. Gel blots were probed with anti-GST or anti-MBP antibody. The full scans of the gel blots (d,e) are shown inSupplementary Fig. 4. (f) The TPL DNA binding on the promoters ofCPDandDWF4are enhanced by BR treatment. TPL DNA-binding was determined by ChIP assay usingTPLp::TPL-HAtransgenic plants. One-week seedlings grown on the medium containing 2 μM PPZ were treated with mock (M) or 100 nM BL for 4 h before crosslinking. Error bars indicate the s.d. (n=3) and **P<0.01 by Student’st-test. Figure 4: BZR1 interacts with TOPLESS through the EAR motif. ( a ) A yeast two-hybrid assay shows the interaction between BZR1 and TPL. Yeast clones were grown on the synthetic dropout (+His) or synthetic dropout without histidine (-His) plus 50 mM 3AT medium. ( b ) Mutation in the EAR motif abolishes the BZR1–TPL interaction. Core Leu residues of the EAR motif were substituted to Ala. Yeast clones were grown on the synthetic dropout (+His) or synthetic dropout without histidine (−His) plus 1 mM 3AT medium. ( c ) BZR1 interacts with TPL and other TPRs. Yeast clones were grown on the synthetic dropout (+His) or synthetic dropout without histidine (−His) plus 5 mM 3AT medium. TPL-N, N-terminal domain of TPL (1–344); TPR1-N, 1–343; TPR2-N, 1–335; TPR3-N, 1–335; and TPR4-N, 1–344. ( d ) BZR1 interacts with TPL through EAR motif in vivo . Arabidopsis mesophyll protoplasts were transfected with TPL-Myc together with bzr1-1D-GFP or bzr1-1DΔEAR-GFP , and the extracted proteins were immunoprecipitated by anti-GFP antibody. Gel blots were probed with anti-Myc or anti-GFP antibody. ( e ) TPL binds to DWF4 promoter through BZR1. GST-TPL-N (amino acids 1–344) was incubated with a biotin-labelled DWF4 promoter DNA (400 bps) together with MBP or MBP-BZR1 and pulled down with streptavidin agarose beads. Gel blots were probed with anti-GST or anti-MBP antibody. The full scans of the gel blots ( d , e ) are shown in Supplementary Fig. 4 . ( f ) The TPL DNA binding on the promoters of CPD and DWF4 are enhanced by BR treatment. TPL DNA-binding was determined by ChIP assay using TPLp::TPL-HA transgenic plants. One-week seedlings grown on the medium containing 2 μM PPZ were treated with mock (M) or 100 nM BL for 4 h before crosslinking. Error bars indicate the s.d. ( n =3) and ** P <0.01 by Student’s t -test. Full size image TPL is not a DNA-binding protein, but it is usually recruited to specific promoter DNA through interaction with DNA-binding transcription factors. To test whether BZR1 recruits TPL to the promoters of BZR1 target genes, we first carried out DNA pull-down assays with a biotin-labelled DWF4 promoter. As expected, TPL was pulled down by the DWF4 promoter DNA only in the presence of BZR1 but not when BZR1 was absent ( Fig. 4e ). Next, we carried out chromatin immunoprecipitation (ChIP) assays using the transgenic plants expressing TPL-HA driven by the native TPL promoter, to test the TPL binding to the promoters of BZR1 targets in vivo . Consistent with the results of the DNA pull-down assays, TPL is associated with the promoters of BZR1-repressed genes ( DWF4 and CPD ) in vivo and the TPL binding to these promoters was enhanced by BR treatment ( Fig. 4f ), which is known to induce BZR1 DNA binding [5] . TPL also bound to the promoters of BR-activated genes ( SAUR15 and IAA19 ), but unlike the binding to DWF4 and CPD promoters the TPL binding to SAUR15 and IAA19 promoters was not enhanced by BR treatment ( Fig. 4f ). TPL is likely to be also recruited to these promoters through other BR-independent transcription factors, such as the AUX/IAA proteins, which also interact with TPL and mediate auxin-responsive expression of SAUR15 and IAA19 (refs 27 , 30 ). Together, these results indicate that through its EAR motif, BZR1 recruits TPL to the promoters of BR-repressed genes. TPL is required for BR responses To further verify the requirement of TPL/TPRs activities in BR responses, we tested the BZR1-repressed genes in the tpl;tpr1;tpr4 triple mutant lacking TPL and two TPR genes [28] . As expected, bzr1-1D caused a much milder repression of CPD and DWF4 in tpl;tpr1;tpr4 than in wild-type background ( Fig. 5a ), supporting that the full TPL/TPRs activities are required for BZR1 repression of these target genes. In contrast, bzr1-1D activation of IAA19 and EXP8 was not significantly affected by the tpl;tpr1;tpr4 mutation, and SAUR15 activation by bzr1-1D was only slightly decreased in tpl;tpr1;tpr4 ( Supplementary Fig. 3 ). These results indicate that TPL/TPRs play a major role in BZR1 repression of target genes but not in BZR1 activation of gene expression. Consistent with the defect in the BZR1 repression of gene expression, the tpl;tpr1;tpr4 seedlings were significantly less sensitive to BR treatment ( Fig. 5b ) in hypocotyl elongation compared with wild type. In addition, the tpl;tpr1;tpr4 triple mutation partially suppressed the PPZ-insensitive phenotypes of the bzr1-1D mutation both in the dark and under light ( Fig. 5c,d ). These results demonstrate that the normal level of TPL/TPR activity is required for BZR1-mediated gene repression and hypocotyl cell elongation. 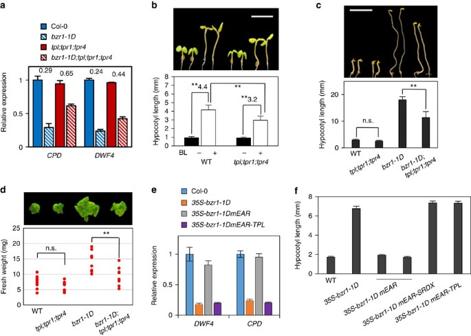Figure 5: TOPLESS is required for BR responses. (a) The BZR1 transcriptional repression activity is compromised intpl;tpr1;tpr4.Total RNA were extracted from etiolated seedlings grown on the medium containing 2 μM PPZ. The relative gene expression levels were determined by qRT–PCR. Numbers indicate the ratios of expression levels (bzr1-1D/Col-0 orbzr1-1D;tpl;tpr1;tpr4/tpl;tpr1;tpr4). Error bars indicate the s.d. (n=3). (b) Thetpl;tpr1;tpr4triple mutant is less sensitive to BR. Seedlings were grown for 5 days on the medium containing either mock or 1,000 nM BL. Numbers indicate ratio of hypocotyl lengths (BL-treated/mock-treated). Error bars indicate the s.d. (n=10 plants) and **P<0.01 by Student’st-test. Scale bar, 5 mm. (c) Thetpl;tpr1;tpr4triple mutation suppresses the long hypocotyl phenotype ofbzr1-1D. Seedlings were grown on the medium containing 2 μM PPZ for 6 days in the dark. Error bars indicate the s.d. (n=10 plants). n.s., not significant and **P<0.01 by Student’st-test. Scale bar, 5 mm. (d) Scatter plot of fresh weight measurements of 3-week-old plants grown on the medium containing 2 μM PPZ. This experiment was repeated with similar results. **P<0.01 by Student’st-test (n=10 plants). (e) TPL fusion at the C terminus restores the transcriptional repression activity of bzr1-1DmEAR. Relative expression fold changes ofCPDandDWF4were determined by qRT–PCR inArabidopsisplants transformed with the indicated constructs, compared with wild type (Col-0). Error bars indicate the s.e. (n=4). (f) TPL fusion restores the activity of bzr1-1DmEAR in promoting hypocotyl elongation. Seedlings were grown in the dark on the medium containing 1 μM BRZ for 5 days. Error bars indicate the s.e. (n=10). Figure 5: TOPLESS is required for BR responses. ( a ) The BZR1 transcriptional repression activity is compromised in tpl;tpr1;tpr4. Total RNA were extracted from etiolated seedlings grown on the medium containing 2 μM PPZ. The relative gene expression levels were determined by qRT–PCR. Numbers indicate the ratios of expression levels ( bzr1-1D /Col-0 or bzr1-1D;tpl;tpr1;tpr4 / tpl;tpr1;tpr4 ). Error bars indicate the s.d. ( n =3). ( b ) The tpl;tpr1;tpr4 triple mutant is less sensitive to BR. Seedlings were grown for 5 days on the medium containing either mock or 1,000 nM BL. Numbers indicate ratio of hypocotyl lengths (BL-treated/mock-treated). Error bars indicate the s.d. ( n =10 plants) and ** P <0.01 by Student’s t -test. Scale bar, 5 mm. ( c ) The tpl;tpr1;tpr4 triple mutation suppresses the long hypocotyl phenotype of bzr1-1D . Seedlings were grown on the medium containing 2 μM PPZ for 6 days in the dark. Error bars indicate the s.d. ( n =10 plants). n.s., not significant and ** P <0.01 by Student’s t -test. Scale bar, 5 mm. ( d ) Scatter plot of fresh weight measurements of 3-week-old plants grown on the medium containing 2 μM PPZ. This experiment was repeated with similar results. ** P <0.01 by Student’s t -test ( n =10 plants). ( e ) TPL fusion at the C terminus restores the transcriptional repression activity of bzr1-1DmEAR. Relative expression fold changes of CPD and DWF4 were determined by qRT–PCR in Arabidopsis plants transformed with the indicated constructs, compared with wild type (Col-0). Error bars indicate the s.e. ( n =4). ( f ) TPL fusion restores the activity of bzr1-1DmEAR in promoting hypocotyl elongation. Seedlings were grown in the dark on the medium containing 1 μM BRZ for 5 days. Error bars indicate the s.e. ( n =10). Full size image The BR-related phenotypes of the tpl;tpr1;tpr4 triple mutant are weaker and likely to be also less specific than typical BR-insenstive mutants, because of genetic redundancy and broad functions of TPL/TPRs as general transcription repressors. To further confirm the essential and sufficient role of the BZR1–TPL interaction in the BR repression of gene expression, we generated transgenic plants overexpressing bzr1-1DmEAR (mutation in the EAR motif) and bzr1-1DmEAR-TPL fusion protein. The mutation of the core Leu residues in the EAR motif (mEAR) abolished the BZR1 interaction with TPL ( Fig. 4b ) and the BZR1 transcriptional repression activities on DWF4 and CPD ( Fig. 5e ). TPL fusion to the C terminus of bzr1-1DmEAR restored the BZR1 transcriptional repression activities ( Fig. 5e ) as well as the hypocotyl promoting activity ( Fig. 5f ), indicating that the TPL recruitment through the EAR motif is necessary and sufficient for these BZR1 functions. TPL/TPRs modulate light sensitivity The BR repression of gene expression has been shown to mediate the BR inhibition of light-induced seedling morphological changes, photomorphogenesis [31] , [32] . BR-activated BZR1 directly binds to the promoters of GATA 4 and BZS1 , which are positive regulators of photomorphogenesis, and represses their expression levels [31] , [32] . As TPL/TPRs are involved in the BZR1 repression of gene expression, we tested whether TPL/TPRs are also required for BZR1 to repress GATA4 and BZS1 . First, we showed, using ChIP assays, that TPL was recruited to the promoters of GATA4 and BZS1 in a BR-dependent manner ( Fig. 6a ). Consistently, BZR1 repression of GATA4 and BZS1 expression was diminished in the tp1;tpr1;tpr4 mutant compared with wild type ( Fig. 6b ). Next, we tested whether loss of TPL/TPRs affects light response of seedlings. 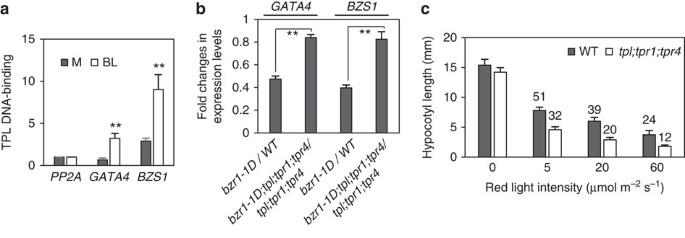Figure 6: TPL/TPRs modulate light sensitivity. (a) TPL binds to the promoters ofGATA4andBZS1in a BR-dependent manner. The TPL-DNA binding was determined by ChIP assay usingTPLp::TPL-HAtransgenic plants. One-week-old seedlings grown on the medium containing 2 μM PPZ were treated with mock (M) or 100 nM BL for 4 h before cross-linking. Error bars indicate the s.d. (n=3) and **P<0.01 by Student’st-test. (b) The BZR1 transcriptional repression ofGATA4andBZS1are compromised in thetpl;tpr1;tpr4triple mutant. Total RNA were extracted from etiolated seedlings grown on the medium containing 2 μM PPZ. The relative expression fold changes ofGATA4andBZS1were determined by qRT–PCR. Error bars indicate the s.d. (n=3) and **P<0.01 by Student's test. (c) Thetpl;tpr1;tpr4seedlings are hypersensitive to red light. Seedlings were grown in various intensities of red light for 5 days. Numbers indicate the percentages of average hypocotyl length relative to that of dark-grown seedling. Error bars indicate the s.d. (n=10). Figure 6c shows that tp1;tpr1;tpr4 is hypersensitive to the red light inhibition of hypocotyl elongation, which is consistent with the high expression levels of GATA4 and BZS1. Together, these results suggest that BZR1–TPL/TPRs interactions modulate the light sensitivity of seedlings through the transcriptional regulation of GATA4 and BZS1 . Figure 6: TPL/TPRs modulate light sensitivity. ( a ) TPL binds to the promoters of GATA4 and BZS1 in a BR-dependent manner. The TPL-DNA binding was determined by ChIP assay using TPLp::TPL-HA transgenic plants. One-week-old seedlings grown on the medium containing 2 μM PPZ were treated with mock (M) or 100 nM BL for 4 h before cross-linking. Error bars indicate the s.d. ( n =3) and ** P <0.01 by Student’s t -test. ( b ) The BZR1 transcriptional repression of GATA4 and BZS1 are compromised in the tpl;tpr1;tpr4 triple mutant. Total RNA were extracted from etiolated seedlings grown on the medium containing 2 μM PPZ. The relative expression fold changes of GATA4 and BZS1 were determined by qRT–PCR. Error bars indicate the s.d. ( n =3) and ** P <0.01 by Student's test. ( c ) The tpl;tpr1;tpr4 seedlings are hypersensitive to red light. Seedlings were grown in various intensities of red light for 5 days. Numbers indicate the percentages of average hypocotyl length relative to that of dark-grown seedling. Error bars indicate the s.d. ( n =10). Full size image HDA mediates BR repression of gene expression The Groucho/TLE-mediated transcription repression has been known to engage HDA [33] . In addition, previous studies have shown that TPL interacts with HDA6 and HDA19 (refs 25 , 28 ), and our proteomic study has identified HDA19 in the BZR1 complex [29] . We confirmed that BZR1 associates with both HDA19 and TPL in vivo ( Fig. 7a ). These results suggested that the HDA activity may be required for the BR repression of gene expression, and thus we tested this hypothesis using a HDA inhibitor Trichostatin A (TSA). Although BR treatment dramatically repressed expression levels of DWF4 and CPD , their expression levels were elevated by TSA treatment and much less affected by BR in the presence of TSA ( Fig. 7b ), indicating that the HDA activity is required for BR repression of gene expression. Consistent with the gene expression pattern, the long-hypocotyl phenotype of bzr1-1D was largely suppressed by the TSA treatment, whereas the wild-type seedlings were much less affected under this condition ( Fig. 7c ). These results support the notion that the BZR1–TPL interaction exploits HDA for the BR repression of gene expression and promotion of cell elongation. 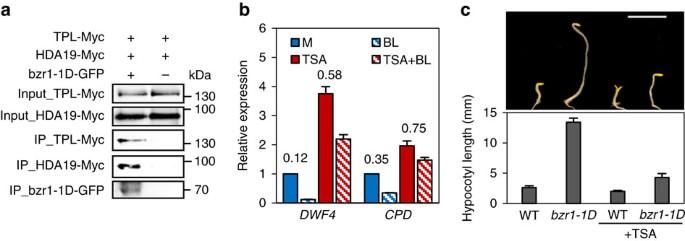Figure 7: BR repression of gene expression requires HDA activity. (a) BZR1 associates with both TPL and HDA19in vivo.Arabidopsismesophyll protoplasts were transfected withbzr1-1D-GFPtogether withTPL-MycandHDA19-Myc, and the extracted proteins were immunoprecipitated by anti-GFP antibody. Gel blots were probed with anti-Myc or anti-GFP antibody. (b) HDA inhibitor, trichostatin A (TSA) diminishes BR repressive effect on the expression ofDWF4andCPD. Total RNA was extracted from 2-week-old plants treated with 100 nM BL±10 μM TSA for 1 h. The relative gene expression levels were determined by qRT–PCR. Error bars indicate the s.d. (n=3). Numbers indicate the ratios of expression levels (BL/M or TSA+BL/TSA). (c) TSA treatment inhibits BZR1 promotion of hypocotyl elongation. Seedlings were grown on the medium containing 2 μM PPZ with or without 1 μM TSA in the dark. The error bars in the lower graph indicate the s.d. (n=10 plants). Scale bar, 5 mm. Figure 7: BR repression of gene expression requires HDA activity. ( a ) BZR1 associates with both TPL and HDA19 in vivo . Arabidopsis mesophyll protoplasts were transfected with bzr1-1D-GFP together with TPL-Myc and HDA19-Myc , and the extracted proteins were immunoprecipitated by anti-GFP antibody. Gel blots were probed with anti-Myc or anti-GFP antibody. ( b ) HDA inhibitor, trichostatin A (TSA) diminishes BR repressive effect on the expression of DWF4 and CPD . Total RNA was extracted from 2-week-old plants treated with 100 nM BL±10 μM TSA for 1 h. The relative gene expression levels were determined by qRT–PCR. Error bars indicate the s.d. ( n =3). Numbers indicate the ratios of expression levels (BL/M or TSA+BL/TSA). ( c ) TSA treatment inhibits BZR1 promotion of hypocotyl elongation. Seedlings were grown on the medium containing 2 μM PPZ with or without 1 μM TSA in the dark. The error bars in the lower graph indicate the s.d. ( n =10 plants). Scale bar, 5 mm. Full size image BZR1 directly represses the expression of TPL and TPRs The genome-wide analyses of BZR1 direct targets showed that TPL and TPRs are direct targets of BZR1 ( Fig. 8a ) [15] . We performed independent ChIP assays using transgenic plants expressing bzr1-1D-CFP under the control of native BZR1 promoter ( BZR1p::bzr1-1D-CFP ). Consistent with the ChIP-Seq result, the promoter regions of TPL , TPR1 , TPR2 and TPR3 were significantly enriched by the BZR1 ChIP compared with the negative control PP2A and UBC30 promoter regions ( Fig. 8b ), confirming that BZR1 binds to these TPL/TPR promoters. BR treatment reduced the expression level of TPR3 by twofold, TPL by ~40% and TPR1 slightly, but had no significant effect on TPR2 expression ( Fig. 8c ), which correlate with their relative binding by BZR1 detected by ChIP–qPCR ( Fig. 8b ). These results suggest that BZR1 mediates repression of TPL and at least two TPRs . In addition, BZR1 repression of TPR3 also requires TPL/TPRs activities, as the expression level of TPR3 was elevated and much less repressed by bzr1-1D in the tpl;tpr1;tpr4 mutant background ( Fig. 8d ), suggesting that BZR1–TPL/TPRs interactions mediate a feedback repression of many members of the TPL/TPR gene family. 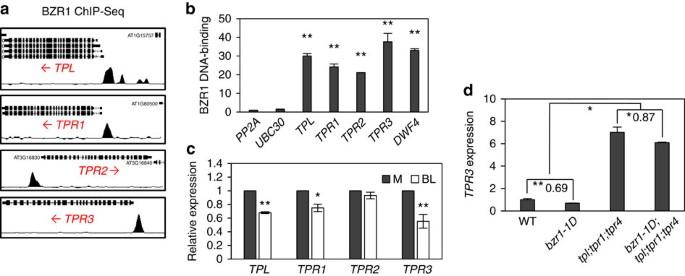Figure 8: BZR1 represses the expression ofTPLandTPRs. (a) ChIP-Seq analyses shows BZR1 binding on the promoters ofTPLandTPRs. Arrows indicate the direction of transcription. (b) ChIP assays confirm that BZR1 binds to promoters ofTPLandTPRs. Transgenic plants expressingbzr1-1D-CFPfrom the nativeBZR1promoter were used for the ChIP assays. BZR1-bound DNA was immunoprecipitated using anti-GFP antibody and analysed by qPCR. BZR1 DNA binding was calculated as the ratio betweenbzr1-1D-CFPand wild-type samples, normalized to that ofPP2A. (c) The expression levels ofTPLandTPR3are reduced by BR treatment. Seedlings grown on the medium containing 2 μM PPZ medium for 7 days were treated with mock (M) or 100 nM BL for 4 h. (d)TPR3repression by BZR1 requires TPL/TPR activity. Total RNA were extracted from etiolated seedlings grown on the medium containing 2 μM PPZ. The relative gene expression levels were determined by qRT–PCR. Numbers indicate the ratios of expression levels (bzr1-1D/Col-0 orbzr1-1D;tpl;tpr1;tpr4/tpl;tpr1;tpr4). The error bars inb–dindicate the s.d. (n=3). **P<0.01 and *P<0.05 by Student’st-test. Figure 8: BZR1 represses the expression of TPL and TPRs . ( a ) ChIP-Seq analyses shows BZR1 binding on the promoters of TPL and TPRs . Arrows indicate the direction of transcription. ( b ) ChIP assays confirm that BZR1 binds to promoters of TPL and TPRs . Transgenic plants expressing bzr1-1D-CFP from the native BZR1 promoter were used for the ChIP assays. BZR1-bound DNA was immunoprecipitated using anti-GFP antibody and analysed by qPCR. BZR1 DNA binding was calculated as the ratio between bzr1-1D-CFP and wild-type samples, normalized to that of PP2A . ( c ) The expression levels of TPL and TPR3 are reduced by BR treatment. Seedlings grown on the medium containing 2 μM PPZ medium for 7 days were treated with mock (M) or 100 nM BL for 4 h. ( d ) TPR3 repression by BZR1 requires TPL/TPR activity. Total RNA were extracted from etiolated seedlings grown on the medium containing 2 μM PPZ. The relative gene expression levels were determined by qRT–PCR. Numbers indicate the ratios of expression levels ( bzr1-1D /Col-0 or bzr1-1D;tpl;tpr1;tpr4 / tpl;tpr1;tpr4 ). The error bars in b – d indicate the s.d. ( n =3). ** P <0.01 and * P <0.05 by Student’s t -test. Full size image BZR1 is a master transcription factor in BR signallling pathway and regulates expression of thousands of genes to elicit various BR responses [15] . Although BR signalling pathway upstream of BZR1 has been relatively well characterized, the molecular mechanism underlying BZR1 regulation of gene expression is still poorly understood. Here we show that the EAR motif at the C terminus of BZR1 is essential for BZR1 regulation of transcription and plant growth, and the EAR motif mediates BR/BZR1 repression of gene expression by recruiting the co-repressor TPL and HDAs. EAR motifs of several plant transcription factors have been shown to act as a transcription repression domain by recruiting the Groucho/TLE-like transcriptional corepressor TPL [34] . We found the EAR motif is highly conserved in the BZR1 family of transcription factors across land plants and it plays a central role in BZR1’s transcriptional functions. Specific deletion or mutations of the EAR motif abolished BZR1’s abilities to regulate gene expression and a wide range of developmental processes, demonstrating an essential role of the EAR motif in BZR1 function. The series in vitro and in vivo experiments demonstrated that the EAR motif of BZR1 mediates interaction with TPL. The BZR1–TPL interaction was detected in yeast two-hybrid, co-IP and in vitro pull-down assays. TPL was also identified as a component of the BZR1 complex by affinity purification followed by mass spectrometry analyses [29] . Deletion of the EAR motif abolished the interaction in both yeast two-hybrid and co-IP assays. Both in vitro DNA-binding assays and ChIP assays demonstrated that BZR1 recruits TPL to the promoters of BR-repressed genes. The essential role for TPL/TPRs in BR repression of gene expression is supported by several lines of evidence. First, BZR1 showed significantly reduced ability to repress several BR-repressed genes in the triple tpl;tpr1;tpr4 mutant compared with wild-type plants. The weak phenotypes of the tpl;tpr1;tpr4 mutant are likely to be due to redundant functions of other members of the TPL/TPR family, as TPR3 expression is increased in the tpl;tpr1;tpr4 mutant and yeast two-hybrid assays indicated that BZR1 interacts with all four TPRs. Second, the TPL fusion to the bzr1-1DmEAR restored the defect of bzr1-1DmEAR in repressing gene expression and promoting hypocotyl elongation, demonstrating that BZR1 interaction with TPL is essential and sufficient for repressing gene expression and promoting cell elongation. Furthermore, TPL and three TPR genes are direct targets of BZR1, and three of them are repressed by BR treatment under our conditions, supporting complex roles of TPL/TPRs in BR responses. Given that TPL/TPRs are positive regulators in BR responses, the transcriptional repression of TPL / TPRs by BZR1 would provide a negative feedback loop that enables fine-tuning the BR responses. Furthermore, as the BZR1-mediated repression requires TPL/TPRs proteins, this creates another feedback loop that helps maintain the cellular level of TPL/TPRs. As TPL/TPRs are exploited by multiple hormonal and developmental pathways (auxin, jasmonic acid, abscisic acid and ethylene) to repress gene expression [26] , [27] , [28] , [35] , [36] , [37] , regulation of TPL/TPRs expression levels by BZR1 potentially allows BR/BZR1 to modulate other signalling pathways. Therefore, TPL/TPRs play important roles in BR responses not only as the transcription repressors of specific BR target genes but also as BR target genes themselves that potentially mediate feedback regulation of BZR1 function and modulate broader secondary gene expression responses. The TPL-induced transcriptional repression has been reported to be at least partly mediated by HDA [34] . A role of HDA in the BZR1 repression of gene expression is supported by the effect of HDA inhibitor TSA on bzr1-1D repression of CPD and DWF4 expression, and BZR1 association with both TPL and HDA19 in vivo . Together, these results demonstrate that BZR1 recruits TPL and HDA to the BR-repressed promoters to mediate transcriptional repression through chromatin modification. The transcriptional repression activity of BZR1 is important not only for feedback regulation of BR homeostasis but also for BR promotion of plant growth [5] . As essential components for BZR1-mediated transcriptional repression, TPL/TPRs play a key role in the biological functions of BR. In addition to the BR biosynthetic genes, two BR-repressed genes encoding positive regulators of photomorphogenesis, GATA4 and BZS1 (refs 31 , 32 ), showed BR-induced TPL promoter binding and TPL/TPR-dependent transcriptional repression. Consistent with TPL/TPR’s function in BZR1-mediated repression of GATA4 and BZS1 , the triple tpl;tpr1;tpr4 mutant showed not only reduced sensitivity to BR treatment but also increased sensitivity to red light treatment in hypocotyl elongation, which indicate that TPL/TPRs play an important role in BR regulation of growth and photomorphogenesis. The function of TPL in BR promotion of growth is further confirmed by the recovery of growth promoting activity of bzr1-1DmEAR with TPL fusion. Together, these results provide strong evidence supporting a central role for the TPL-mediated transcriptional repression activity of BZR1 in BR regulation of cell elongation and photomorphogenesis, as well as in the feedback inhibition of BR biosynthesis. Although the EAR motif has been shown to mediate transcription repression in several plant transcription factors as well as in BZR1, our study provides evidence that the EAR motif of BZR1 may also mediate transcriptional activation. First, the expression of BZR1 direct target genes that are activated by BR and bzr1-1D were not activated by bzr1-1DΔEAR in transgenic plants. Second, when bzr1-1DΔEAR-GR was induced to translocate to the nucleus, the expression level of SAUR15 was not increased, in contrast to bzr1-1D-GR that significantly activated SAUR15 expression. Third, bzr1-1DΔEAR did not activate the PRE5 promoter activity in the transient gene expression assay. Last, the artificial SRDX domain recovered the defect in transcriptional activation of bzr1-1DΔEAR. SRDX contains a different EAR motif from that of BZR1 (LDLDLELRLGFA instead of LELTL), and thus the results suggest that the loss of activation function in bzr1-1DΔEAR is due to the loss of the EAR motif rather than another overlapping domain. The EAR motif exists in a large number of transcription factors and whether the EAR motif can mediate transcription activation in other factors is an important question to be answered in future studies. Our observation also cautions the interpretation of results obtained with SRDX fusion transcription factors. How the transcriptional activation and repression activities of BZR1 are determined? Apparently, the cis -elements of the promoter specify BZR1’s transcriptional activity by probably recruiting different co-factors. A recent study showed that a MYB transcription factor MYBL2 is a transcription repressor and interacts with BZR2/BES1 (ref. 20 ). Interestingly, MYBL2 has an internal LxLxL motif [35] but instead uses a C-terminal TLLLFR motif for transcription repression [38] . Nevertheless, MYBL2 was identified as a TPL-interacting protein in the yeast two-hybrid screen [35] and thus it is possible that MYBL2 stabilizes BZR1/BZR2 interactions with TPL and thereby enhances transcriptional repression. Another BZR2/BES1-interacting transcription factor HAT1 also represses gene expression, but loss-of-function hat1;hat2 mutant showed normal fold change of BR-responsive gene expression [21] , and thus HAT1 appears not essential for BZR2/BES1 transcriptional repression. Alternatively, transcriptional repression might be the default activity of BZR1 in the absence of co-activator that blocks the EAR motif, as suggested by the repression of artificial promoter by the BZR1 fusion to the LexA DNA-binding domain [5] . It is conceivable that the EAR motif in BZR1 must be blocked and inaccessible to TPL at the promoter to be activated by BZR1. Consistent with this notion, BR treatment increased TPL association with BR-repressed promoters but not BR-activated promoters. It is possible that the EAR motif in BZR1 is involved in interaction with co-activators at the BR-activated promoters, to both mediate gene activation and prevent recruitment of TPL repressor. BZR1 activation of transcription appears to involve interaction with bHLH factors. Both BZR1 and BZR2/BES1 interact with bHLH factors of the PIF family [16] , and their shared target genes are significantly more likely to be activated than repressed by BR. BZR2/BES1 has also been shown to interact with another bHLH factor BIM1 and histone-modifying enzymes to mediate the transcriptional activation [13] , [17] , [19] . Whether the EAR motif of BZR1 is involved in the interactions with these co-transcription activators remains to be determined in future studies. Transcription factors with dual functions of activation and repression are common in both plants and animals. For example, WUSCHEL activates AGAMOUS expression but represses the expression of ARR6 and ARR7 (ref. 39 ). In metazoan, the T-cell factor (TCF) transcription factors mediate both repression and activation of target gene expression. When the Wnt signalling pathway is off, TCF interacts with Groucho/TLE corepressor to repress its target genes. Wnt signalling inactivates GSK3, leading to accumulation of β-catenin in the nucleus; β-catenin displaces Groucho/TLE from TCF and re-assembles a transcription activator complex, switching from repression to activation [40] . In this case, TCF bound to the same promoter is switched from a repressor to an activator by exchange of interacting proteins. The mode of action of BZR1 appears more similar to that of dorsal, which represses some target genes by recruiting Groucho/TLE but interacts with the bHLH factor twist to activate target genes that contain twist-binding sites [41] , [42] , [43] . Unlike BZR1’s EAR motif, which is required for both repression and activation, the Groucho/TLE-interaction domain at the C terminus of dorsal is required for transcription repression but not activation. It seems that BZR1 shares features of repressor displacement with TCF, cis -element-dependent co-activator interaction with dorsal and inactivation by GSK3 with β-catenin. Furthermore, both BZR1 and dorsal are targets of leucine-rich repeat receptor-mediated signalling pathways [2] , [3] . Therefore, the BR signalling pathway shares striking similarities with the Wnt and Toll pathways of metazoan, while mechanistic details seem to have evolved to provide appropriate efficiency required for the different levels of developmental plasticity of the organisms. Plant materials and growth conditions Arabidopsis thaliana plants were grown in a greenhouse with a 16-h light/8-h dark cycle at 22–24 °C for general growth and seed harvesting. All the plants used in this study are in Col-0 ecotype background. The tpl;tpr1;tpr3 triple mutant was provided by Zhang and coworkers [28] . The TPLp::TPL-HA plants used for ChIP assay was provided by Somers and coworkers [25] . Constructs The full-length complementary DNA of bzr1-1D (also bzr1-1DΔEAR ) was fused to GR by overlapping PCR. The resulting bzr1-1D-GR and bzr1-1DdEAR-GR were inserted into pENTR/SD/D-TOPO vector (Invitrogen) and subcloned into gateway compatible pEarleyGate101 vector for transformation into Arabidopsis . For the Arabidopsis mesophyll protoplast transfections, the full-length cDNA of TPL and HDA19 (without stop codon) was cloned into the gateway-compatible pGWB17 plasmid, and the cDNA (without stop codon) of bzr1-1D and bzr1-1DΔEAR was cloned into the gateway-compatible pEarleyGate101 plasmid. The full-length cDNA of bzr1-1D (BZR1P234L ) and bzr1-1DmEAR ( bzr1-1D L328/330A ) were cloned into plant expression vectors under the control of the 35S C4PPDK promoter as previously reported [10] , [44] . All mutants of BZR1 were generated using the QuickChange Site-Directed Mutagenesis kit (Stratagene) according to the manufacturer’s instructions. To generate bzr1-1DmEAR-SRDX- and bzr1-1DmEAR-TPL -overexpressing transgenic lines, the SRDX sequence and full-length cDNA of TPL were tagged to bzr1-1DmEAR at the C terminus region and sub-cloned into a plant expression binary vector, pCB302ES [44] . Hypocotyl and root length measurements Sterilized seeds by 70% (v/v) ethanol and 0.01% (v/v) Triton X-100 were plated on MS medium (PhytoTechnology Laboratories) supplemented with 0.75% phytoagar. After 3 days of incubation at 4 °C, seedlings were irradiated by white light for 6 h to promote germination and then incubated in specific conditions for 5–7 days. Seedlings were photocopied and hypocotyl and root lengths were measured by using ImageJ software ( http://rsb.info.nih.gov/ij ). Arabidopsis protoplast isolation and transfection Leaves from 4-week-old plants grown in the short photoperiod were cut to 0.5–1 mm leaf strips and digested by enzyme solution (1.5% cellulase R10; 0.4% macerozyme R10; 0.4 M mannitol; 20 mM KCl; 20 mM MES at pH 5.7; 10 mM CaCl 2; 0.1% BSA) for 3 h at room temperature after being vacuum infiltrated for 30 min in the dark. The enzyme/protoplast solution was diluted by an equal volume of W5 buffer (154 mM NaCl; 125 mM CaCl 2 ; 5 mM KCl; 5 mM glucose; 2 mM MES at pH 5.7). The enzyme solution containing protoplast was filtered through 75-μm nylon mesh and the protoplasts were collected by centrifugation at 100 g for 1 min. After washing with W5 solution, the protoplasts were resuspended with W5 solution and incubated on ice for 30 min. After removing W5 by centrifugation at 100 g for 30 s, the protoplasts were resuspended with MMG solution (0.4 M mannitol; 15 mM MgCl 2 ; 4 mM MES at pH 5.7). For DNA transfection, an equal volume of PEG buffer (40% PEG4000; 0.2 M mannitol; 0.1 M Ca(NO 3 ) 2 ) was mixed with the protoplasts and DNA, and four volumes of W5 buffer were added to stop the transfection after 15 min. The resulting solution was mixed well by gently inverting the tube and the protoplasts were pelleted by centrifugation at 100 g for 1 min. The transfected protoplasts were resuspended gently in 0.5 ml of WI solution (0.5 M mannitol; 20 mM KCl; 4 mM MES at pH 5.7) and cultured under weak light at room temperature overnight. Co-immunoprecipitation assays About 2 × 10 4 isolated Arabidopsis mesophyll protoplast were transfected with a total 20 μg of DNA and incubated overnight. Total proteins were extracted from the protoplasts using the IP buffer (50 mM Tris-Cl pH7.5, 1 mM EDTA, 75 mM NaCl, 0.1% Triton X-100, 5% glycerol, 1 mM phenylmethyl sulphonyl fluoride, 1 × Protease Inhibitor). After centrifugation at 20,000 g for 10 min, supernatants were incubated for 1 h with 5 μg of polyclonal anti-YFP antibody (custom-made) immobilized on protein A/G agarose beads. The beads were then washed for three times with 1 ml of IP buffer and eluted samples were analysed by immunoblotting using Anti-Myc (Cell Signaling Technology, mouse mAb, 1:5,000 dilution) and Anti-GFP (Clontech JL-8, mouse mAb, 1:5,000 dilution) antibodies. Transient gene expression assays Isolated Arabidopsis mesophyll protoplasts (2 × 10 4 ) were transfected with a total 20 μg of DNA and incubated overnight. Protoplasts were harvested by centrifugation and lysed in 50 μl of passive lysis buffer (Promega). Firefly and Renilla (as an internal standard) luciferase activities were measured by using a dual-luciferase reporter kit (Promega). The reporter promoters (1 kb of CPD promoter and 1.5 kb of PRE5 promoter) were cloned upstream of the firefly luciferase gene in pGreen–0800II–luc vector, which also contains the 35S promoter— Renilla luciferase gene. Statistic significance was determined by Student’s t -test. qRT–PCR gene expression analysis Total RNA was extracted by using the Spectrum Plant Total RNA kit (Sigma). M-MLV reverse transcriptase (Fermentas) was used to synthesize cDNA from the RNA. Quantitative real-time RT–PCR was performed in LightCycler 480 (Roche). PP2A was used to as an internal control. Gene-specific primers are listed in Supplementary Table 1 . Chromatin immunoprecipitation assays The plants grown under white light for 2 weeks or in the dark for 5 days were harvested and cross-linked for 20 min in 1% formaldehyde under vacuum. The chromatin complex was isolated, resuspended in lysis buffer (50 mM Tris–HCl pH 8.0, 10 mM EDTA, 200 mM NaCl, 0.5% Triton X-100, 1 mM phenylmethyl sulphonyl fluoride) and sheared by sonication to reduce the average DNA fragment size to around 500 bps. The sonicated chromatin complex was immunoprecipitated by affinity-purified polyclonal anti-YFP antibodies (5 μg, custom-made) or anti-HA antibody (Roche; 3F10), which was incubated with protein A agarose/salmon DNA (Millipore) overnight. The beads were washed with low-salt buffer (50 mM Tris–HCl at pH 8.0, 2 mM EDTA, 150 mM NaCl, 0.5% Triton X-100), high-salt buffer (50 mM Tris-HCl at pH 8.0, 2 mM EDTA, 500 mM NaCl, 0.5% Triton X-100), LiCl buffer (10 mM Tris-HCl at pH 8.0, 1 mM EDTA, 0.25 M LiCl, 0.5% NP-40, 0.5% deoxycholate) and TE buffer (10 mM Tris-HCl at pH 8.0, 1 mM EDTA), and eluted with elution buffer (1% SDS, 0.1 M NaHCO 3 ). After reverse cross-linking, the DNA was purified with a PCR purification kit (Thermo Scientific) and analysed by ChIP–qPCR. Enrichment of DNA was calculated as the ratio between transgenic plants and wild-type control, normalized to that of the PP2A coding region as an internal control. Statistical significance was determined by Student’s t -test. Primers for qPCR are listed in Supplementary Table 1 . DNA pull-down assays GST-TPL-N (amino acids 1–344 of TPL cloned into pDEST15 vector), MBP and MBP-BZR1 ( pMAL-C2 ) proteins were expressed in BL21 codon plus Escherichia coli cells and purified either using glutathione beads (GE Healthcare) or amylose resin (NEB) according to manufacturer’s protocols. The DWF4 promoter fragment was amplified by PCR using the biotin-labelled primers ( Supplementary Table 1 ). GST-TPL-N was incubated with the biotin-labelled DNA together with MBP or MBP-BZR1 protein, and then DNA-binding proteins were pulled down by streptavidin agarose beads (Sigma) and analysed by immunoblotting. How to cite this article: Oh, E. et al. TOPLESS mediates brassinosteroid-induced transcriptional repression through interaction with BZR1. Nat. Commun. 5:4140 doi: 10.1038/ncomms5140 (2014).